Non-uniform membrane diffusion enables steady-state cell polarization via vesicular trafficking Actin-based vesicular trafficking of Cdc42, leading to a polarized concentration of the GTPase, has been implicated in cell polarization, but it was recently debated whether this mechanism allows stable maintenance of cell polarity. Here we show that endocytosis and exocytosis are spatially segregated in the polar plasma membrane, with sites of exocytosis correlating with microdomains of higher concentration and slower diffusion of Cdc42 compared with surrounding regions. Numerical simulations using experimentally obtained diffusion coefficients and trafficking geometry revealed that non-uniform membrane diffusion of Cdc42 in fact enables temporally sustained cell polarity. We show further that phosphatidylserine, a phospholipid recently found to be crucial for cell polarity, is enriched in Cdc42 microdomains. Weakening a potential interaction between phosphatidylserine and Cdc42 enhances Cdc42 diffusion in the microdomains but impedes the strength of polarization. These findings demonstrate a critical role for membrane microdomains in vesicular trafficking-mediated cell polarity. The actin cytoskeleton and vesicular trafficking have crucial roles in cell polarization in a variety of systems from mammalian epithelial cells and Drosophila oocytes to plant pollen tubes [1] , [2] , [3] . The Rho-family GTPase Cdc42 is a highly conserved regulator of cytoskeleton organization and cell polarity [4] . A mechanism of cell polarization identified in the budding yeast Saccharomyces cerevisiae entails a positive feedback loop between Cdc42-stimulated actin assembly and actomyosin-based vesicular trafficking of Cdc42 (refs 5 , 6 ), which results in spontaneous symmetry breaking and concentration of Cdc42 to a small patch of the plasma membrane (PM) at one end of the cell, often referred to as the polar cap. The polar cap marks the site for cell surface growth that leads to bud or shmoo formation [7] , and its maintenance is facilitated by active endocytic recycling to counter membrane diffusion of Cdc42 (refs 8 , 9 ). An analytical model with the assumption of balanced Cdc42 flux and mass conservation demonstrated the existence of a steady-state solution for this system of cell polarity [8] , [9] . However, a surprising finding was reported in a recent study with a discrete simulation of Cdc42 trafficking that considered not only the protein dynamics but also insertion and excision of membrane patches through exocytic and endocytic events, respectively [10] . The simulations showed that in order for vesicular trafficking to establish a polar cap of Cdc42, Cdc42 must be concentrated on exocytic vesicles relative to the internal source membrane. However, even under this condition, the model predicted that continued vesicle trafficking would deplete the internal pool over time. At this stage polarized exocytosis would dilute Cdc42 in the PM due to continual membrane insertion with low Cdc42 concentration, eventually leading to a dissipated polar cap. This result implies the implausibility of a stable polarized state through the vesicle trafficking-based mechanism. In considering the dramatic difference in theoretical predictions with or without the discrete account of membrane dynamics and conservation, we reasoned that it was possible that crucial details were unknown and thus unaccounted for in the discrete model depicting exocytic and endocytic events. To this end, we performed dual-colour confocal imaging using a highly sensitive single-photon detector to investigate the spatiotemporal relationship between the dynamic Cdc42 distribution and the sites of endocytosis and exocytosis. To restrict our investigation to the membrane-based mechanism for polarized localization of Cdc42, experiments were performed in Δrdi1 cells, lacking the yeast guanine nucleotide dissociation inhibitor. In this mutant background Cdc42 does not exchange rapidly between the cytosol and membrane compartments and cell polarity is actin dependent [9] . In other words, this work addresses solely the feasibility of cell polarization through actin-based membrane trafficking, but not a redundant, cytosolic Cdc42 targeting pathway [6] , [11] , [12] . Here we present evidence not only that endocytosis and exocytosis of Cdc42 occur in spatially separate regions of the PM but also that Cdc42 diffusion in these regions is considerably different, resulting in microdomains with locally concentrated Cdc42. Contributing to Cdc42’s slow diffusion in specific areas is the phospholipid phosphatidylserine (PS), which has been shown to be trafficked with secretory vesicles in yeast and is required for robust cell polarity [13] . Modelling and experimental analyses demonstrate that these features, especially non-uniform Cdc42 diffusion, have important roles in stable maintenance of cell polarity via membrane-based recycling. Spatial organization of Cdc42 at the PM To determine the spatial organization of Cdc42 recycling at the PM, we first imaged GFP-Cdc42 with mCherry-tagged Myo5, which marks the sites of endocytosis immediately before endocytic internalization [14] . As expected endocytic patches are in general concentrated in the polar cap region, as demonstrated by a time series projection ( Fig. 1 , Supplementary Fig. S1 ). By confocal imaging using a highly sensitive detector (avalanche photodiode (APD)), instantaneous localization of Cdc42 within the polar cap was found to be heterogeneous, and exhibited dynamic and discrete puncta within the polar cap. Imaging with total internal reflection fluorescence (TIRF) microscopy showed these Cdc42 puncta to be associated with the PM rather than internal membrane structures close to the PM such as the cortical ER ( Supplementary Fig. S2a ). Upon subtraction of the time-averaged membrane distribution, discrete fluctuations in protein levels along the PM became even more apparent ( Fig. 1a , Supplementary Fig. S1a ). Interestingly, the Cdc42 puncta are spatially and temporally anti-correlated with the dynamic endocytic patches labelled with Myo5-mCherry ( Fig. 1a ). The anti-correlated distribution of GFP-Cdc42 and Myo5-mCherry was also confirmed by using TIRF microscopy ( Supplementary Fig. S2b ). Note that because Myo5 disappears from the endocytic patch just before vesicle internalization [14] , the observed low concentration of Cdc42 at Myo5 patches was not a consequence of endocytosis. 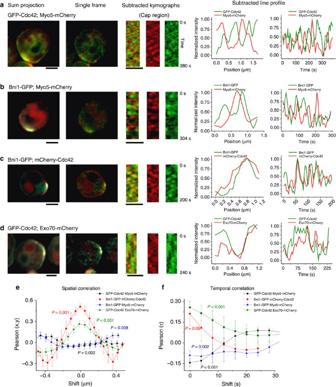Figure 1: Spatial organization of endocytic and exocytic domains relative to Cdc42 distribution. (a–d) Left most column shows representative time-summed images of the localization of the indicated proteins. These images show the overall presence of the analysed proteins in the polar cap. The column second from the left shows example single time point images showing punctate appearance of the proteins observed. The three columns that follow show sum-subtracted kymographs (merged followed by mCherry and GFP) of the polar cap region from image series showing anti-correlated (a,b) or correlated (c,d) fluctuations of the two proteins in each pair as indicated. Raw (non-average subtracted) kymographs are shown inSupplementary Fig. S1. The second from right plot shows an example fluorescence profile at a single time point from the kymographs to the left, whereas the right most graph shows a time trace at a single cortical location. Scale bars, 2 μm. Average Pearson cross-correlation between red and green fluorescence spatially (along rows of the kymographs) (e) and temporally (columns of kymographs) (f). Negative correlation was observed for Bni1 with Myo5, and Cdc42 with Myo5, whereas positive correlation was observed between Bni1 and Cdc42, and Exo70 and Cdc42 at small space (e) or time shifts (f). Plots show mean and s.e.m. from 6 to 8 kymographs per pair.P-values are based on a one-component Student’st-test, compared with zero, or a random distribution. Figure 1: Spatial organization of endocytic and exocytic domains relative to Cdc42 distribution. ( a – d ) Left most column shows representative time-summed images of the localization of the indicated proteins. These images show the overall presence of the analysed proteins in the polar cap. The column second from the left shows example single time point images showing punctate appearance of the proteins observed. The three columns that follow show sum-subtracted kymographs (merged followed by mCherry and GFP) of the polar cap region from image series showing anti-correlated ( a , b ) or correlated ( c , d ) fluctuations of the two proteins in each pair as indicated. Raw (non-average subtracted) kymographs are shown in Supplementary Fig. S1 . The second from right plot shows an example fluorescence profile at a single time point from the kymographs to the left, whereas the right most graph shows a time trace at a single cortical location. Scale bars, 2 μm. Average Pearson cross-correlation between red and green fluorescence spatially (along rows of the kymographs) ( e ) and temporally (columns of kymographs) ( f ). Negative correlation was observed for Bni1 with Myo5, and Cdc42 with Myo5, whereas positive correlation was observed between Bni1 and Cdc42, and Exo70 and Cdc42 at small space ( e ) or time shifts ( f ). Plots show mean and s.e.m. from 6 to 8 kymographs per pair. P -values are based on a one-component Student’s t -test, compared with zero, or a random distribution. Full size image By using the same analysis as above, spatial and temporal anti-correlation were also observed between Myo5-mCherry and Bni1-GFP, which marks the ends of actin cables in the polar cap region and presumed sites of exocytosis [15] ( Fig. 1b ). By contrast, strong positive spatial and temporal correlation of mCherry-Cdc42 with Bni1-GFP was observed ( Fig. 1c ). Confirming the co-localization of Cdc42 puncta with sites of exocytosis, strong positive correlation was also observed in RDI1 cells ( Supplementary Fig. S3 ) and between GFP-Cdc42 and Exo70-mCherry, a member of the exocyst complex [16] , [17] ( Fig. 1d–f ). These results reveal the existence of two types of regions within the polar cap: regions of high Cdc42 concentration (referred to as Cdc42 puncta) correlating with sites of exocytic vesicle delivery, surrounded by regions in the polar cap with relatively low concentration of Cdc42 where sites of endocytosis are preferentially located. The Cdc42 puncta do not appear to distinguish between the active (GTP-bound) or inactive (GDP-bound) form of Cdc42, and show positive correlation with the distribution of the Cdc42 guanine nucleotide exchange factor Cdc24, suggesting that Cdc42 can be locally activated within the puncta ( Supplementary Fig. S3 ). Non-uniform membrane diffusion of Cdc42 It was surprising to find that Cdc42 displays a punctate distribution and remains concentrated at the sites of exocytic delivery, given its reported, fairly rapid overall diffusion coefficient in the PM [8] . One possible explanation is that the regions with high or low Cdc42 concentrations have different Cdc42 diffusion coefficients, leading to a heterogeneous distribution. To test this, we performed inverse fluorescence recovery after photobleaching (iFRAP) experiments. In iFRAP, a region of the cell is photobleached, and loss of fluorescence is monitored in an adjacent (unbleached) region to reveal dynamics of removal of protein from the unbleached area. We used iFRAP to observe the dissipation of the polar cap through diffusion following bleaching of the cytosolic pool and the membrane outside the polar cap ( Fig. 2a ). To avoid complication from Cdc42 recycling via actin-dependent exocytosis and endocytosis, this analysis was done immediately following treatment with Latrunculin A (LatA) to block Cdc42 recycling in the Δrdi1 background. Little overall fluorescence was lost from the PM during the duration of the iFRAP measurement, confirming that loss of intensity from the unbleached region was due to membrane diffusion, not cytosolic recycling (data not shown, see Methods ). Membrane kymographs from the iFRAP experiments revealed that the Cdc42 puncta no longer moved laterally in the membrane, consistent with stoppage of endocytic patch movement in the presence of LatA [18] . 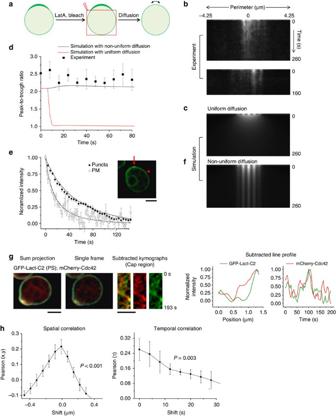Figure 2: Cdc42 exhibits different diffusion properties in distinct regions of the plasma membrane. (a) Experimental scheme for observing Cdc42 diffusion in the PM by iFRAP (inverse FRAP) analysis. (b) Two representative kymographs showing the decay of GFP-Cdc42 fluorescence in the polar cap following bleaching of the cytosol and surrounding membrane inΔrdi1cells treated with LatA. Cells were examined shortly after LatA treatment while the polar cap was still intact. (c) Simulation of the decay of the Cdc42 polar cap in the above iFRAP experiment with a uniform diffusion coefficient of 0.013 μm2s−1. (d) Comparison of the simulated evolution of peak-to-trough ratios (defined as the ratio of Cdc42 intensity in puncta to that in-between puncta) during an iFRAP experiment assuming uniform or non-uniform diffusion with that observed experimentally. (e) Average fluorescence decay curves from iFRAP measurements at puncta (arrow in the inset image;n=17) or a PM location close to but outside the polar cap (arrowhead in the inset image;n=28). Smooth black lines represent the simulated decay profiles from which the slow and fast diffusion coefficients were obtained (seeMethods). (f) Simulated iFRAP kymograph based on an initial heterogeneous distribution and two different diffusion coefficients as determined ine. (g) A sum projection image, single time point image, and subtracted kymographs for the PS marker, GFP-Lact-C2, and mCherry-Cdc42. Representative subtracted line profiles in position and time are shown to the right, as described inFig. 1. (h) Average spatial and temporal correlations for GFP-Lact-C2 and mCherry-Cdc42 as inFig. 1e. Scale bars, 2 μm. Figure 2: Cdc42 exhibits different diffusion properties in distinct regions of the plasma membrane. ( a ) Experimental scheme for observing Cdc42 diffusion in the PM by iFRAP (inverse FRAP) analysis. ( b ) Two representative kymographs showing the decay of GFP-Cdc42 fluorescence in the polar cap following bleaching of the cytosol and surrounding membrane in Δrdi1 cells treated with LatA. Cells were examined shortly after LatA treatment while the polar cap was still intact. ( c ) Simulation of the decay of the Cdc42 polar cap in the above iFRAP experiment with a uniform diffusion coefficient of 0.013 μm 2 s −1 . ( d ) Comparison of the simulated evolution of peak-to-trough ratios (defined as the ratio of Cdc42 intensity in puncta to that in-between puncta) during an iFRAP experiment assuming uniform or non-uniform diffusion with that observed experimentally. ( e ) Average fluorescence decay curves from iFRAP measurements at puncta (arrow in the inset image; n =17) or a PM location close to but outside the polar cap (arrowhead in the inset image; n =28). Smooth black lines represent the simulated decay profiles from which the slow and fast diffusion coefficients were obtained (see Methods ). ( f ) Simulated iFRAP kymograph based on an initial heterogeneous distribution and two different diffusion coefficients as determined in e . ( g ) A sum projection image, single time point image, and subtracted kymographs for the PS marker, GFP-Lact-C2, and mCherry-Cdc42. Representative subtracted line profiles in position and time are shown to the right, as described in Fig. 1 . ( h ) Average spatial and temporal correlations for GFP-Lact-C2 and mCherry-Cdc42 as in Fig. 1e . Scale bars, 2 μm. Full size image Particularly noticeable was the fact that the Cdc42 puncta persisted for 60–90 s after photobleaching the cytosol and surrounding membrane ( Fig. 2b ). Numerical simulation of the iFRAP experiment using a single apparent diffusion coefficient of 0.013 μm 2 s −1 , based on the average iFRAP decay rate and geometry (see Methods ), matches the experimental decay time; however, with uniform diffusion, the simulation predicts that the heterogeneous initial distribution would rapidly equilibrate with surrounding regions ( Fig. 2c ). This was clearly contrary to what was observed experimentally ( Fig. 2b ). To quantitatively compare the experimental observation with model simulations, we calculated the evolution of the peak-to-trough ratio, or the ratio of Cdc42 intensity in puncta to that in-between puncta (see Supplementary Fig. S4 ), as a function of time in the iFRAP experiment. With uniform diffusion, the peak-to-trough ratio was predicted to decay rapidly to a value of 1 within ~10 s ( Fig. 2d ). By contrast, the experimentally observed peak-to-trough ratio remained constant throughout the time frame of the experiment (over 80 s, Fig. 2d ), suggesting that the observed Cdc42 diffusion was inconsistent with having a uniform diffusion coefficient throughout the PM. To directly assess the existence of non-uniform diffusion of Cdc42 in the PM, we compared the kinetics of fluorescence decay between Cdc42 puncta and non-puncta regions adjacent to the polar cap in iFRAP experiments. A dramatic difference in fluorescence decay profiles was indeed observed ( Fig. 2e ). The decay profile outside the puncta is consistent with a diffusion coefficient of 0.053 μm 2 s −1 , supporting the conclusion of heterogeneous diffusion. To model the iFRAP data more accurately, we fixed the diffusion coefficient away from the puncta and varied the size, shape and diffusion coefficient of the puncta region to match the experimental decay time and peak-to-trough ratios. Modelling of the iFRAP data with the diffusion coefficient profile shown in Supplementary Fig. S6 led to an estimated membrane diffusion coefficient of 0.0061 μm 2 s −1 at the puncta ( Fig. 2e ) (see Methods for model details). Simulation of iFRAP experiments using these two different diffusion coefficients gave rise to peak-to-trough ratios that closely resembled the experimentally observed values ( Supplementary Fig. S6 ) and persisted throughout the experimental time frame, validating the assumption of two non-identical diffusion coefficients for Cdc42 at and away from the puncta ( Fig. 2d ). Two well-characterized microdomains are known to exist in the yeast PM and include the membrane compartment of Pma1 (MCP) and the membrane compartment of Can1 (MCC) [19] , [20] . However, we found no overlap of Pma1-mCherry or Pil1-mCherry, a marker for the MCC [20] , with sites of Cdc42 enrichment ( Supplementary Fig. S5 ). Pma1-mCherry, in particular, was completely absent from areas of polarized growth (where GFP-Cdc42 is preferentially localized); this was not due to relatively slow mCherry maturation as the same observation was made with Pma1-GFP alongside mCherry-Cdc42 ( Supplementary Fig. S5 ). Recent studies reported that PS is delivered to the polar cap via secretory vesicles and has an important role in Cdc42 localization, possibly through interaction between the negatively charged head group of PS and a polycationic peptide near the COOH terminus of Cdc42 (refs 13 , 21 ). It was conceivable that the regions of slow Cdc42 diffusion correlate with microdomains where PS is accumulated. Indeed, when membrane kymographs were compared between the PS biosensor GFP-Lact-C2 [13] , [21] , [22] (refs 13 , 21 , 22 ) and mCherry-Cdc42, high spatial and temporal cross-correlation was observed ( Fig. 2h , compared with Fig. 1 ). Reducing the potential charge interaction between Cdc42 and PS with the cdc42 S185D mutation [21] led to faster diffusion in the puncta ( Supplementary Fig. S4c ) and reduced Cdc42 concentration in the microdomains, as indicated by a reduced peak-to-trough ratio in the polar cap ( Supplementary Fig. S4a ). Modelling of this data gave a Cdc42 S185D diffusion coefficient at the puncta of 0.022 μm 2 s −1 (see Methods ), more than three times faster than that for wild-type Cdc42. iFRAP of GFP-Lact-C2 following LatA treatment showed slow diffusion ( Supplementary Fig. S4d ), consistent with reports of slow diffusion of other phospholipids in the yeast PM [23] . These data suggest that the Cdc42 puncta may be explained by biased diffusion towards membrane microdomains that are enriched for PS. Simulations of Cdc42 polarity establishment With the above details in the spatial organization of Cdc42 trafficking and diffusion, we performed discrete numerical simulations of Cdc42 polar cap formation and maintenance. First, we implemented the exact model in the recent work [10] . Discrete simulations were performed assuming a flat, circular membrane with a predefined membrane area to which Cdc42-containing exocytic vesicles are delivered (see Supplementary Methods and Supplementary Fig. S6 for description of simulations). Upon vesicle docking, the exocytic membrane is inserted into the PM along with its cargo such as Cdc42. The PM is then expanded isotropically to accommodate the added area, and diffusion serves to redistribute Cdc42 along the PM. The material and membrane area associated with the exocytic vesicle are removed from a well-mixed internal membrane compartment. Endocytosis is accomplished by isotropically invaginating the membrane, leading to loss of Cdc42 and surface area from the PM. Simulations assuming uniform diffusion and spatially merged endocytosis and exocytosis confirmed the previous conclusion that without Cdc42 concentrating on vesicles, exocytosis does not lead to polarization ( Fig. 3b ), and that concentration of Cdc42 on secretory vesicles allowed initial formation of a weak polar cap that diminished rapidly ( Fig. 3c ). A slower but uniform diffusion coefficient at a value consistent with the average iFRAP decay rate enhanced the strength and duration of polarity but was still insufficient for achieving a stable polarized state ( Fig. 3d ). 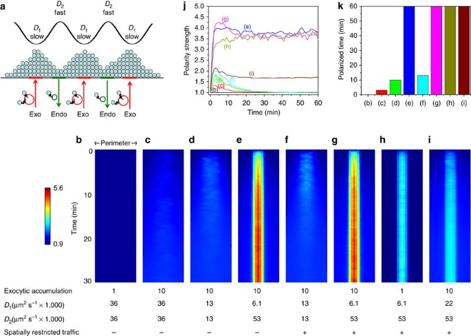Figure 3: Numerical simulation of Cdc42 polarization under various conditions. (a) Cartoon representation of the relative spatial organization of endocytosis and exocytosis and non-uniform diffusion in the polar cap region. Blue balls represent Cdc42 molecules. Red and green circles depict exocytic (exo) and endocytic (endo) vesicles, respectively. (b–i) Simulations of Cdc42 polarization with assumptions similar to those used previously (b–d)10(that is, uniform diffusion and spatially merged endocytosis and exocytosis) and with geometric factors observed in this study (e–i). Descriptions for each condition are given underneathb–i, including the different diffusion coefficients, exocytic vesicle Cdc42 enrichment and spatial relationship of endocytosis and exocytosis used in each simulation. Exocytic accumulation refers to the enrichment of Cdc42 on secretory vesicles compared with internal membrane. (j,k) Quantification of polarity strength as a function of time (j), defined as the ratio of maximum/minimum Cdc42 concentration over the entire cell periphery, colour coded to match the quantification of polarity duration ink, defined as the time during which polarity strength is above 1.3, for the simulations shown inb–i. Figure 3: Numerical simulation of Cdc42 polarization under various conditions. ( a ) Cartoon representation of the relative spatial organization of endocytosis and exocytosis and non-uniform diffusion in the polar cap region. Blue balls represent Cdc42 molecules. Red and green circles depict exocytic (exo) and endocytic (endo) vesicles, respectively. ( b – i ) Simulations of Cdc42 polarization with assumptions similar to those used previously ( b – d ) [10] (that is, uniform diffusion and spatially merged endocytosis and exocytosis) and with geometric factors observed in this study ( e – i ). Descriptions for each condition are given underneath b – i , including the different diffusion coefficients, exocytic vesicle Cdc42 enrichment and spatial relationship of endocytosis and exocytosis used in each simulation. Exocytic accumulation refers to the enrichment of Cdc42 on secretory vesicles compared with internal membrane. ( j , k ) Quantification of polarity strength as a function of time ( j ), defined as the ratio of maximum/minimum Cdc42 concentration over the entire cell periphery, colour coded to match the quantification of polarity duration in k , defined as the time during which polarity strength is above 1.3, for the simulations shown in b – i . Full size image Strikingly, the incorporation of two different Cdc42 diffusion coefficients as estimated following the geometry observed experimentally ( Fig. 3a ) was sufficient to produce a stable polar cap lasting >60 min, well beyond the time span of the yeast polarized growth phase ( Fig. 3e ). Conceptually, the presence of microdomains with slower diffusion than the surrounding areas helps to concentrate Cdc42 even when the internal pool is being depleted. The incorporation of spatially separate endocytic and exocytic sites did not lead to sustainable polar cap in the absence of non-uniform diffusion ( Fig. 3f ), but resulted in slightly stronger initial polar cap formation when added to the model with non-uniform diffusion ( Fig. 3g ). As a test case, we modelled the polarization of the Cdc42 S185D mutant assuming that D 2 (off-puncta diffusion) is the same as wild-type Cdc42 (see Methods ) while using a D 1 (at-puncta diffusion) value of 0.022 μm 2 s −1 (see above). Despite the reduced diffusion non-uniformity for this mutant, the model predicts that a polarized distribution could be obtained ( Fig. 3i ) but the resulting steady-state polarity strength, defined as the ratio of maximum/minimum Cdc42 concentration over the entire cell periphery, would be greatly compromised ( Fig. 3j ), qualitatively consistent with the diminished polarity strength observed for Cdc42 S185D ( Supplementary Fig. S4b , see below for quantitative validation of this prediction). FCS analysis of cytosolic Cdc42 Another prediction of the previous model [10] was that in order for Cdc42 to polarize initially, Cdc42 must concentrate strongly on secretory vesicles compared with internal membrane and PM [10] . However, the concentration of Cdc42 on vesicles in yeast cells has been difficult to determine by conventional imaging because of the small size of the vesicles (80–100 nm), their mobility in the cytosol and the presence of a considerable non-vesicle-bound pool. Thus, to estimate Cdc42 concentration on vesicles, we used fluorescence correlation spectroscopy (FCS), which is uniquely able to determine the stoichiometry of proteins in mobile fractions in live cells [24] . The average molecular brightness of GFP-Cdc42 was higher than that of the monomer control, suggesting that at least one diffusing pool of Cdc42 had a stoichiometry higher than 1 ( Fig. 4a ; (see Methods ). As previously shown in wild-type cells [21] , the autocorrelation profile of GFP-Cdc42 in the Δrdi1 background did not fit to a single-component diffusion model but instead fit well to a two-component diffusion model ( Fig. 4b ) ( P <0.001), with the fast and slow species having cytosolic diffusion coefficients of 3.4±1.7 and 0.10±0.1 μm 2 s −1 , respectively. Whereas the fast diffusion coefficient was close to that expected for a small soluble Cdc42 species, perhaps unprenylated Cdc42, the slow one may be due to a vesicle-bound pool. In support of this conclusion, the cdc42 C188S mutation, which eliminates the prenylation site [25] , had a drastically diminished slow pool ( Supplementary Fig. S7a ), whereas the sec6-4 mutant that accumulates secretory vesicles at the restrictive temperature [26] , [27] had an enhanced amplitude of the slowly diffusing species ( Supplementary Fig. S7b ). By contrast, the relative amplitude of the slow pool was not diminished in an arp3-2 mutant, which blocks endocytosis at the restrictive temperature ( Supplementary Fig. S7c ). Furthermore, the diffusion coefficient of the slow pool was consistent with an average stokes radius of 50–100 nm based on free diffusion model (see Methods ), consistent with the known size of exocytic vesicles but not the much smaller endocytic vesicles [28] , [29] . 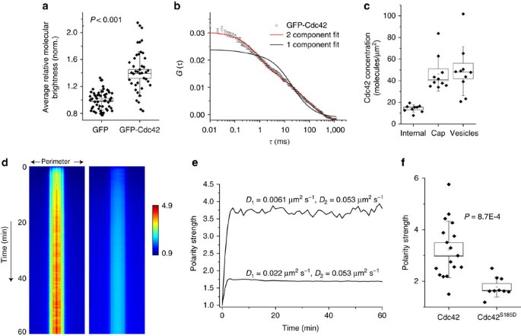Figure 4: Numerical simulation of Cdc42 polarization using measured concentrations. (a) Average molecular brightness of mobile GFP-Cdc42 in polarized, unbuddedΔrdi1cells compared with a cytosolic GFP control. In each box plot the small box shows the mean, line shows median, large box the s.e.m. and whiskers show s.d. (b) Average autocorrelation decay of GFP-Cdc42 inΔrdi1fitted with 1-component or 2-component models for free three-dimensional diffusion (note these are different from the models used to simulate two-dimensional membrane diffusion of Cdc42 on the PM inFig. 2). (c) Calibrated imaging was used to compare the concentration of GFP-Cdc42 on exocytic vesicles (from FCS analysis) to the GFP-Cdc42 concentration at formed polar caps. Internal membrane concentration was estimated as the concentration on PM in non-polarized cells (see text for explanation). Box plots presented as ina. (d) Simulated kymograph for polar cap formation that included non-uniform diffusion for Cdc42 (left panel,D1=0.0061 μm2s−1;D2=0.053 μm2s−1) and Cdc42S185D(right panel,D1=0.022 μm2s−1;D2=0.053 μm2s−1) and 3.4-fold enrichment of Cdc42 onto exocytic vesicles as determined by FCS and calibrated imaging. (e) Polarity strength (as explained inFig. 3jlegend) as a function of time from the simulations ind. (f) Comparison of experimental polarity strength between wild type and mutant (seeSupplementary Methods). Box plots are as described ina. Figure 4: Numerical simulation of Cdc42 polarization using measured concentrations. ( a ) Average molecular brightness of mobile GFP-Cdc42 in polarized, unbudded Δrdi1 cells compared with a cytosolic GFP control. In each box plot the small box shows the mean, line shows median, large box the s.e.m. and whiskers show s.d. ( b ) Average autocorrelation decay of GFP-Cdc42 in Δrdi1 fitted with 1-component or 2-component models for free three-dimensional diffusion (note these are different from the models used to simulate two-dimensional membrane diffusion of Cdc42 on the PM in Fig. 2 ). ( c ) Calibrated imaging was used to compare the concentration of GFP-Cdc42 on exocytic vesicles (from FCS analysis) to the GFP-Cdc42 concentration at formed polar caps. Internal membrane concentration was estimated as the concentration on PM in non-polarized cells (see text for explanation). Box plots presented as in a . ( d ) Simulated kymograph for polar cap formation that included non-uniform diffusion for Cdc42 (left panel, D 1 =0.0061 μm 2 s −1 ; D 2 =0.053 μm 2 s −1 ) and Cdc42 S185D (right panel, D 1 =0.022 μm 2 s −1 ; D 2 =0.053 μm 2 s −1 ) and 3.4-fold enrichment of Cdc42 onto exocytic vesicles as determined by FCS and calibrated imaging. ( e ) Polarity strength (as explained in Fig. 3j legend) as a function of time from the simulations in d . ( f ) Comparison of experimental polarity strength between wild type and mutant (see Supplementary Methods ). Box plots are as described in a . Full size image To determine whether the ‘fast’ pool represents monomeric Cdc42, we examined cross-correlation between GFP-Cdc42 and mCherry-Cdc42. Cross-correlation was observed between GFP-Cdc42 and mCherry-Cdc42 with a slow, not fast, transit time ( Supplementary Information ; Supplementary Fig. S7d ), suggesting that the fast pool of Cdc42 was monomeric, whereas at least a fraction of the slow diffusing pool contained multiple Cdc42 molecules per mobile particle. We fixed the brightness of the fast pool to that of monomer green fluorescent protein (GFP), and freely fit the brightness of the slow pool (see Methods ), which yielded an average stoichiometry of Cdc42 in the slow pool of 1.5±0.2 proteins per particle or a concentration of 49±7 molecules μm −2 on vesicles of 100 nm diameter ( Fig. 4c , Supplementary Information ) [29] , [30] . By using calibrated imaging (see Methods ), we determined the average concentration of Cdc42 at the polar cap to be 46±5 molecules μm −2 ( Fig. 4c ). Fluorescence lifetime imaging verified that GFP has a similar lifetime freely diffusing in the cytosol as it does bound to either cytosolic Cdc42 or membrane-bound Cdc42 ( Supplementary Fig. S7e ), therefore fluorescence intensity is an accurate measure of relative protein abundance. Before cell polarization, where Cdc42 concentration is likely in equilibrium between the PM and internal membrane, the Cdc42 concentration at the PM was measured to be 14±1 molecules μm −2 , ~3.4 times lower than that at the polar cap or the concentration on exocytic vesicles in polarized cells ( Fig. 4c ). Simulation of the model with a 3.4 × concentration of Cdc42 on secretory vesicles coupled with non-uniform diffusion and segregated endocytosis and exocytosis on the PM showed long-lasting and stable polar caps ( Fig. 4d ). The predicted polarity strength agreed well with that observed experimentally for both wild-type Cdc42 and Cdc42 S185D ( Fig. 4f ). Interestingly, our model predicts the presence of non-uniform diffusion to be sufficient for prolonged polarity even in the absence of Cdc42 accumulation on secretory vesicles (assuming equal concentrations between secretory vesicles and internal membranes) ( Fig. 3h ), although in this case it takes slightly longer to reach the steady-state polarity strength ( Fig. 3j ). In addition, in the case of a reduction in non-uniform diffusion (something that could happen in nascent caps or under environmental perturbation), concentration of Cdc42 onto exocytic vesicles allows for increased polarity strength ( Supplementary Fig. S8a ). Given the stability of the polar cap in the discrete simulations, we revisited the presence of a polarized steady state with an analytical model by incorporating non-uniform diffusion using a simple geometry that represents exocytosis in a central region with slower diffusion than the rest of the PM, and endocytosis outside this region ( Supplementary Methods ; Supplementary Fig. S6b–d ). A polarized steady-state solution was indeed found. By contrast, no significant steady-state polarization was obtained given uniform Cdc42 diffusion ( Supplementary Fig. S6e–g ). A role for actin and actin-based vesicular trafficking in driving cell polarization was first revealed in an experimental system, where overexpression of constitutively active Cdc42 leads to spontaneous polarization of G1-arrested yeast cells [5] . Subsequent studies demonstrated that during normal cell polarization at the start of bud formation, the actin-mediated mechanism functions in parallel with a pathway that relies on the adaptor protein Bem1 (ref. 11 ) and that both pathways are required for achieving a signal-responsive and robust polarized state [9] , [12] , [31] . Mechanistic details by which these pathways drive cell polarization remain elusive. Mathematical modelling provides a powerful tool for quantitative exploration of conceptual models derived from experimental evidence [32] . Failure of a model to predict the expected outcome is indicative of crucial gaps in our understanding based on which model assumptions are made. The results described in this study demonstrate that for the actin/membrane trafficking-based mechanism to achieve a stable polarized state with simultaneous balance of protein and membrane flux, Cdc42 diffusion in the PM must be non-uniform with the presence of microdomains towards which Cdc42 diffusion is biased. Previous work demonstrated that membrane proteins in yeast diffuse more slowly than their counterparts in mammalian cells and that if the diffusion is slow enough, recycling through endocytosis would be sufficient to polarize the proteins [33] . We found in this study that although overall slow diffusion enhances temporary polarization, it is the non-uniformity of Cdc42 diffusion that allows sustained polarization. Our findings may be of particular importance to the polarization of mammalian cells where overall membrane diffusion is more rapid. Lateral segregation into distinct, coexisting microdomains has recently been reported as a widely occurring phenomenon for PM-associated proteins in yeast [34] . It is proposed that self-assembly of these microdomains is an emergent outcome of multiple weak interactions between proteins and lipids. The possible role for Cdc42–PS interaction in determining Cdc42 localization and mobility is reminiscent of early work on electrostatic interactions of PS with the myristylated protein, MARCKS. A polycationic region near the N-terminal myristate lipid anchor was postulated to be surrounded by negatively charged PS, causing a ‘lipid shell’ that may also recruit additional lipids [35] . Interestingly, this contributes to a punctate appearance of MARCKS, in which MARCKS co-localizes with proteins such as F-actin and talin [36] , [37] . We speculate that a similar mechanism may contribute to the formation of Cdc42 microdomains, which are also rich for the formin family actin nucleator Bni1. A role for PS in Cdc42 microdomain formation and the crucial requirement for these microdomains in Cdc42 polarization are consistent with the recent finding that Cdc42 polarizes extremely poorly in the cho1 mutant deficient in PS synthesis [13] . Aside from PS, the Cdc42 microdomains, which can harbour either GTP- or GDP-bound Cdc42, are also enriched for proteins such as Bni1, Exo70 and Cdc24. All three proteins are capable of direct interaction with Cdc42 (refs 38 , 39 , 40 , 41 ), and Exo70 and Cdc24 also contain lipid-binding motifs [41] , [42] , [43] . Our observation of two apparent diffusion coefficients for Cdc42 does not conflict with the possibility that the slow apparent diffusion is due to Cdc42 binding and dissociating from other components of the microdomains. Whereas Cdc24 governs Cdc42 activation, Bni1 and Exo70 are key effectors mediating downstream actin nucleation and exocytosis. Thus, the Cdc42 microdomains may not only result from multiple protein–protein and protein–lipid interactions but also represent centres of Cdc42 signalling in the establishment of cell polarity. In Supplementary Information , we also entertained a model of concentration-dependent diffusion with Cdc42 concentration inversely related to its own diffusion coefficient but found this model unable to recapitulate the microdomain dynamics ( Supplementary Fig. S8d ). On the basis of the evidence presented, we favour a model where targeted delivery of Cdc42 through vesicle trafficking is accompanied by the deposition of lipid components, such as PS, which help to provide an initial Cdc42 diffusion trap. Interaction of Cdc42 with Cdc24 leads to Cdc42 activation, accompanied by additional recruitment of Cdc24 through Cdc42 effectors such as Cla4 and Bem1, as previously proposed [44] . Further recruitment of the Cdc42 effectors such as Bni1 and Exo70 (or Sec3) (ref. 41 ) not only mediates localized actin cable assembly and vesicle exocytosis but also re-enforces the microdomains that slow Cdc42 diffusion through additional protein and lipid interactions. Although the presence of non-uniform diffusion remedies the issue of unstable polarity predicted by a model based on a set of simple assumptions [10] , our findings do not rule out other potential mechanisms that can contribute to polarity maintenance. For example, a ring of septins appears around the polar cap just minutes after initial Cdc42 polarization [45] . The septin ring serves as a diffusion barrier to restrict lateral diffusion of Cdc42 (refs 46 , 47 ) and could prevent the potential decline of polarity strength. In addition, whereas the simplest assumption posits Cdc42 protein flux balance to be accompanied by membrane conservation, this coupling may not be obligatory due to the presence of multiple pathways for membrane trafficking and recycling [1] . In conclusion, membrane microdomains have been studied extensively in many cellular systems [34] , [35] , [48] and have been implicated in GTPase signaling [49] , [50] . The results presented in this study not only demonstrate the theoretical feasibility of vesicular trafficking to achieve a stable polarized state but also predict a critical role for membrane microdomains in this process by modulating the diffusion properties of a master polarity regulator. As such, the macroscopic organization of the cell may originate in part from microscopic self-organization of protein–membrane complexes. Yeast culture and drug treatment Yeast strains used in this study are listed in Supplementary Table S1 . Yeast cells were grown in synthetic complete media to mid-log phase before analysis. For the iFRAP experiments with LatA (BioMol), 50 μM LatA was added immediately before data acquisition. In most experiments, GFP-Cdc42 was controlled under the CDC42 promoter [9] ; however, for GFP-Cdc42 S185D , GFP-Cdc42 C188S and GFP-Cdc42 R66E in the arp3-2 mutant, and GFP-Cdc42 in the sec6-4 mutants, the inducible GAL1 promoter was used to drive GFP-Cdc42 expression. In these experiments, the GAL1 promoter was turned on with galactose for 90–120 min. At this induction time, the induced expression of Cdc42 proteins was at a level similar to the expression level using the CDC42 promoter [9] . The functionality of the tagged proteins was previously validated in the strain background of S288c [9] , [14] , [16] , [51] . Generation of membrane kymographs Two-colour time-lapse movies were acquired using the APD imaging module of a Zeiss Confocor 3. The 488- and 561-nm laser lines were used to excite GFP and mCherry, respectively, and emission was collected through BP 505–540 and LP 580 filters. Before kymograph generation, images were spatially binned 2 × 2 to result in a pixel size of ~80 nm, and kymographs were generated in ImageJ. Using custom built plugins in ImageJ, the average profiles in space and time were subtracted before correlation to eliminate photobleaching and retain only fluctuations in membrane concentrations (and not the overall cap profile). A pinhole of 1.5–1.8 airy units was used, and images were acquired with either 2 or 4 s time resolution. Average spatial and temporal Pearson product-moment correlations functions were generated using the following equations [52] : Here cov a [ x , y ] is the covariance of x and y variables over either the spatial coordinate ( a = x ) or the temporal coordinate ( a = t ) and var a [ x ] is the similarly defined variance. Average correlation curves were generated from between 5 and 7 kymographs, and the P -value compared with zero listed was computed by the one-sample Student’s t -test using OriginPro software. Determination of membrane diffusion of GFP-Cdc42 in Δrdi1 cells from iFRAP experiments To eliminate complications from Cdc42 recycling, Δrdi1 cells were treated with 50 μM LatA, followed immediately by photobleaching of the cytosol and majority of cell membrane (70–90%), and the decay of fluorescence in the unbleached PM region due to membrane diffusion was monitored by time-lapse acquisition using APD detectors. The average decay of the unbleached region was fit to an exponential to determine the characteristic half-time. To ensure that the majority of the loss of localized fluorescence in the iFRAP measurement was due to membrane diffusion, and not internalization, the recovery of the bleached cytosolic protein was monitored, and compared with the whole-cell intensity following the bleach step. The cytosolic increase during the measurement was corrected for geometry, as previously described [9] . Less than 15% of the total membrane fluorescence was lost during the measurement to internalization, whereas the loss of the unbleached region to the surrounding membrane reached 80–90% during the time course of the measurement. These measurements indicate that the decrease in localized membrane intensity in the iFRAP measurement was largely due to membrane diffusion, and not internalization. For determination of the fast diffusion coefficient outside the cap area, iFRAP data was generated outside of the region containing puncta, and fit to get the representative tau value. Simulations were used to determine the diffusion coefficient that matches this tau, given an average unbleached membrane area consisting of 71 μm 2 and a bleach region of circumference 2.6 μm. Given the complex relationship between non-uniform diffusion coefficients with unknown experimental spatial distribution and the fluorescence decay, we chose to use a semi-quantitative parameter matching approach to the iFRAP data analysis to determine the diffusion coefficient of molecules inside the puncta regions. This approach consisted of simulation of a two-dimensional iFRAP experiment with polar cap geometry, similar to that observed experimentally, and 19 regions of reduced diffusion centred on the cap region to emulate the regions of enhanced fluorescence and reduced diffusion observed experimentally ( Fig. 2e , Supplementary Fig. S6 ). The diffusion coefficient in the puncta regions is described as a sum of damped Lorentzians (Lorentzians to the 0.8 power) subtracted from the fast diffusion value. As this function at times exceeds the minimum diffusion coefficient, it is truncated at that value, giving the central puncta a somewhat larger size ( Supplementary Fig. S6 ). The slow diffusion puncta were placed at the distances of 0.62 and 1.2 μm from the centre of the simulation plane. The simulation was carried out with a Gaussian convolution method as described for the more complex trafficking simulation described below, but with a square membrane employing periodic boundary conditions. To expedite the simulations, the diffusion coefficient profile was digitized to 32 values and diffusion probability lookup tables were created for these values before the simulation. The fast diffusion coefficient was estimated with uniform diffusion. The slow diffusion coefficient and the size of the slow diffusion puncta in the simulation were varied to match the experimental peak-to-trough ratio in the prebleached steady state, as well as the experimental half-time of the puncta. This process was repeated iteratively to make sure that scaling the diffusion coefficients did not affect the peak-to-trough ratio significantly. For Cdc42 S185D , membrane localization was reduced to the point where iFRAP data away from the cap could not be obtained reliably. To estimate the diffusion coefficient inside the puncta, we analysed the puncta iFRAP data as described above, with the simplification that D 2 was held the same as for wild-type Cdc42. This resulted in values of 0.022 and 0.053 μm 2 s −1 for D 1 and D 2 , respectively, for a ratio of 2.4. Cytosolic diffusion of GFP-Cdc42 in Δrdi1 cells The diffusion profile of GFP-Cdc42 in Δrdi1 was measured in live yeast cells using FCS as previously described [53] . GFP was excited using the 488-nm laser line of a Zeiss Confocor 3. Emission was sent through a 565-nm dichroic and a BP 505–540-nm filter. APDs were used to collect photons. The autocorrelation decay was calculated using standard methods [53] and fit using a one- and two-component model, with a triplet time of 250 μs. The two-component fit was justified using a standard t -test ( P <0.001). The two-component fit yielded transit times of 2.1±1.1 and 72±9 ms for the fast and slow pool, respectively. FCS determination of concentration of Cdc42 on vesicular structures The amplitude of an FCS curve can be written as a function of the relative number of molecules and molecular brightness: The average intensity obeys the simple relationship: Here ε i and N i are the molecular brightness and average number in the focal volume, respectively, for species i . In this study, two diffusion components for Cdc42 are observed, one that is a monomer and diffuses freely in the cytosol with a short diffusion time, and a second that is composed of vesicles with a Poisson distribution of Cdc42 molecules on them and a slow diffusion time. Given that the above equation is additive, we can write separate equations for the amplitudes of the slow and fast components: Here ε GFP is the molecular brightness of monomeric GFP, n is the vesicle occupancy, is the average vesicle occupancy and γ is a shape factor used in FCS [54] . We can also write an expression for the average intensity: Given the experimentally measureable variables of G (0) fast , G (0) slow , the average intensity and the molecular brightness of ε GFP from observation of a control sample, it is possible to calculate the three unknowns: N fast , N slow and . In the case of free diffusion, the Stokes–Einstein equation predicts an inverse relationship between diffusion coefficient and the hydrodynamic radius. Hence, comparison of diffusion time of something of unknown size to cytosolic GFP, of known size, allows for an estimate of molecular radius of the unknown particle, if a spherical shape is assumed. See Supplementary Information for detailed methods that include TIRF, calibrated imaging, lifetime imaging, numerical simulations and an analytical model. How to cite this article: Slaughter, B. D. et al. Non-uniform membrane diffusion enables steady-state cell polarization via vesicular trafficking. Nat. Commun. 4:1380 doi: 10.1038/ncomms2370 (2013).